Transient-axial-chirality controlled asymmetric rhodium-carbene C(sp2)-H functionalization for the synthesis of chiral fluorenes In catalytic asymmetric reactions, the formation of chiral molecules generally relies on a direct chirality transfer (point or axial chirality) from a chiral catalyst to products in the stereo-determining step. Herein, we disclose a transient-axial-chirality transfer strategy to achieve asymmetric reaction. This method relies on transferring point chirality from the catalyst to a dirhodium carbene intermediate with axial chirality, namely a transient-axial-chirality since this species is an intermediate of the reaction. The transient chirality is then transferred to the final product by C(sp 2 )-H functionalization reaction with exceptionally high enantioselectivity. We also generalize this strategy for the asymmetric cascade reaction involving dual carbene/alkyne metathesis (CAM), a transition-metal-catalyzed method to access chiral 9-aryl fluorene frameworks in high yields with up to 99% ee . Detailed DFT calculations shed light on the mode of the transient-axial-chirality transfer and the detailed mechanism of the CAM reaction. Metal carbene reaction is one of the most versatile methods for the assembly of valuable molecules with structural complexity and diversity [1] , [2] , [3] , [4] , [5] , [6] , [7] , [8] . In this regard, the pursuit of practical and efficient catalytic approach has been of long-standing appealing, especially the catalytic asymmetric carbene transformations, such as cyclopropanation [9] , [10] , X–H insertion [11] , [12] , C–H insertion [13] , [14] , [15] , [16] , hydride migration [17] , cycloaddition [18] , [19] , ylide formation followed by rearrangement [20] or interception [21] , and others [22] , [23] , [24] , [25] , [26] , [27] , [28] . Generally, the asymmetry induction in these metal-carbene reactions heavily relied on the chiral catalyst-associated species, and the asymmetric transfer strategy is a point-to-point chirality transfer manner. For example, the enantioselectivity control in catalytic asymmetric electrophilic aromatic substitution reaction, which happens at the H -shift step, is enabled by the point chirality of the catalyst via a metal-associated zwitterionic intermediate [29] or Wheland-type intermediate [30] (Fig. 1a , path a, MZI , through a M–C single bond). However, in most cases, partially leaving or even dissociation of the metal catalyst could occur to form the free zwitterionic intermediate (Fig. 1a , path b, FZI ), especially in the case with the neutral dirhodium(II) complex [31] , so the subsequent transformation will not secure the high stereoselectivity. Therefore, it is highly challenging and desirable for the development of stereoselective carbene transformations with efficient and practical strategies. Fig. 1: Asymmetry induction in metal-carbene reactions. a Asymmetry induction in catalytic metal-carbene C(sp 2 )-H functionalization. b Chirality in transient carbene intermediate. c This work describes the transient axial-chirality-controlled asymmetric C(sp 2 )–H functionalization. The pink crescent = chiral ligand (L = large group, S = small group). M = metal catalyst. Rh 2 L 4 * = chiral dirhodium complex. Full size image On the other hand, the axial chirality has been found in a variety of rotation-hindered molecules [32] , [33] , [34] , [35] , [36] , [37] , [38] , [39] , such as BINAP and BINOL derivatives, which have been widely used as privileged ligands or catalysts in asymmetric catalysis [40] , [41] , [42] , [43] , [44] , [45] . Inspired by the unique structures of these chiral ligands with axial chirality, we hypothesized that, when the dirhodium complexes catalyze the generation of metal-carbene species with steric bulky carbene precursors, such as ortho -substituted aryl carbene, a transient axial-chirality will be formed in the corresponding carbene intermediate (Fig. 1b ). The axial chirality in the intermediate is called transient axial chirality, considering this chirality will then be transfer to the final product by the followed reaction. In other word, instead of heavily relying on the point chirality of the metal catalyst in the later stereo-determining step (e.g., Fig. 1a ), the final chirality transfer from catalyst to product in this mode would be determined by the initially formed axial chirality between the catalyst and the substrate, due to the restricted rotation of these carbene intermediates in the followed transformations. Thus, high enantioselectivity could be envisioned in metal-carbene reactions based on this transient axial-chirality transfer strategy. Herein, we report our recent results by applying this asymmetric transfer strategy, the asymmetric formal C(sp 2 )-H bond insertion reaction of donor/donor carbene through a transient axial-chirality-induced point chirality strategy, which provides a straightforward access to chiral 9-aryl fluorene frameworks with exceptionally high enantioselectivity (Fig. 1c , reaction 1). Moreover, we generalize this strategy for asymmetric cascade reaction, in which the donor/donor carbene is generated in situ via a dual carbene/alkyne metathesis (CAM) process [46] , [47] , [48] , [49] , [50] , [51] , [52] , [53] , [54] , and directly construction of polycyclic 9-aryl fluorenes with high enantioselectivity (Fig. 1c , reaction 2) [55] , [56] . Considering the chiral fluorenes have found broad applications in various fields, including in pharmaceuticals [57] , photoelectrical materials [58] , and theoretical studies [59] ; the present asymmetric reaction could add complementary values in this respect. 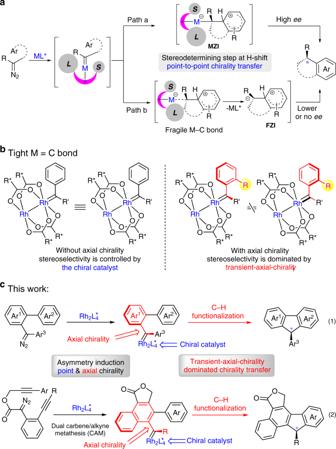Fig. 1: Asymmetry induction in metal-carbene reactions. aAsymmetry induction in catalytic metal-carbene C(sp2)-H functionalization.bChirality in transient carbene intermediate.cThis work describes the transient axial-chirality-controlled asymmetric C(sp2)–H functionalization. The pink crescent = chiral ligand (L = large group, S = small group). M = metal catalyst. Rh2L4* = chiral dirhodium complex. Reaction optimization We began our investigation of the asymmetric C–H functionalization reaction with diaryl diazo compound 1a , which is a typical donor/donor-type carbene precursor, as model substrate (Table 1 ). To optimize reaction conditions, Rh 2 ( S -TCPTTL) 4 was used as the catalyst, and solvents were initially evaluated (entries 1–5), from which we found that reaction in tert -butyl methyl ether (TBME) afforded 2a with the highest selectivity (entry 5, 82% ee and 92% yield). Lowering the reaction temperature did not improve the selectivity (entry 6). Further investigation of a variety of dirhodium complexes turned out that the optimum enhancement was achieved by Rh 2 ( S -TFPTTL) 4 with four electron-withdrawing fluoro substituents on the phthalimide ring (entry 10, 90% yield, 99% ee ). It should be mentioned that slowly addition of the rhodium catalyst to the diazo compound is essential in all these reactions to ensure the high enantioselectivity. Notably, in comparison with the analogous thermal induced version, no Buchner reaction product was observed under current conditions [60] . Table 1 Condition optimization. 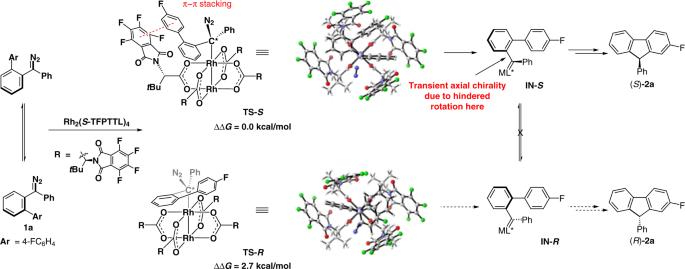Fig. 2: Enantioselectivity transition states of reaction 1 with1ato2aas example. The forming of theS-configuration product2ais the favored one (TS-Sis favored overTS-Rby 2.7 kcal/mol. Calculations at SMD(toluene)-M06L-D3/Def2TZVP//PBE-D3/Def2SVP/W06 level). Full size table Substrate scope With the optimized reaction conditions in hand for reaction 1, the catalytic asymmetric C–H insertion reaction with a variety of substituted diaryl diazo compounds 1 has been tested, and the results are summarized in Table 2 . Unexceptionally, a series of substrates 1a – 1f bearing electron-neutral, -deficient, or -rich substitutions on the aromatic ring react smoothly to give the corresponding products in 90–96% yields with 90–99% ee ( 2a – 2f ). Substrates with 1-naphthyl, 2-fluorophenyl, and 3-fluorophenyl groups are all tolerated under current conditions, delivering the corresponding products in excellent yields and selectivity ( 2g – 2i ). For the detail of the regioselectivity of 2i , see Supplementary Fig. 147 . Substrates with substitutions on the other aryl group do not affect the high reactivity, the corresponding products 2j and 2k are isolated in high yields with 95% and 92% ee , respectively. Table. 2 Substrates scope of direct asymmetric C–H functionalization a . Full size table Considering the limited accessibility and inherent instability of the precursors of the donor/donor-type carbene species, we intend to utilize the carbene/alkyne metathesis reaction for the generation of the analogous carbene intermediate in situ (Fig. 1c , reaction 2). After a brief optimization, polycyclic fluorene product 4a was obtained in 90% yield with 92% ee from the alkyne-tethered propargyl diazoacetate 3a in the presence of 1.0 mol% Rh 2 ( S -TFPTTL) 4 in TBME at 40 °C, and a detrimental effect on the selectivity by increasing the amounts of the chiral rhodium complex has been observed in this case (see Supplementary Table 1 for details). It is worth mentioning that the only catalyst involved in this four-step cascade transformation is a chiral dirhodium catalyst; and this catalyst is responsible for the observed asymmetry induction with high enantiocontrol in this carbene/alkyne metathesis-aromatic substitution cascade reaction [46] , [47] , [48] , [49] , [50] , [51] , [52] , [53] . The ( R )-configuration of the generated chiral center in the 9-aryl fluorene is confirmed by single-crystal X-ray diffraction analysis of its chloro-derivative 4b , and the configurations of other compounds are assigned by analogy. 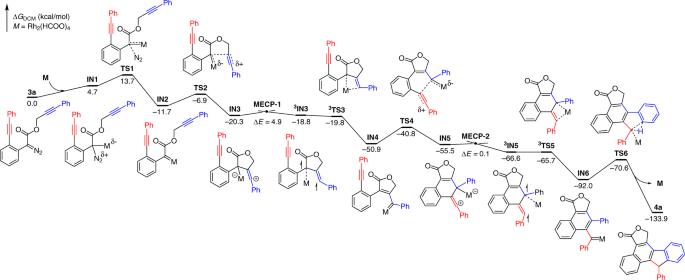Fig. 3: Gibbs energy profile for catalytic cascade reaction 2 with3ato4aas example. The discovery of carbene–Rh-dimer complex formation via ISC process in CAM process. Calculations at SMD(DCM)-M06L/6-311G(d,p)&SDD//PBE/6-31G(d)&SDD level). MECP minimum energy-crossing point. Then, the generality of this cascade reaction with a variety of alkyne-tethered diazo compounds 3a–3u was tested with the optimized reaction conditions (Table 3 ). A series of substrates 3a – 3f bearing electron-neutral, -deficient, or -rich substitutions on the terminating aromatic ring reacted smoothly to give the corresponding products in 63–90% yields with high to excellent enantioselectivity ( 4a – 4f ), and 99% ee was observed with CF 3 -substituted product 4d . The donor/donor carbene intermediate that generated via two carbene/alkyne metathesis process provides a valuable tool for the complement of the selective carbene transformations [61] , which indicates that a different asymmetry induction/transfer model could be involved in this catalytic reaction. Reaction with meta -substituted material 3 g led to the preferential formation of sterically less encumbered 4 g in 53% yield with 97% ee , concomitant with a small amount of 4 g’ in 60% ee (see Supplementary Fig. 147 for detail). On the other hand, the ortho -substituted diazo compound 3 h was found to have very low reactivity, which was caused by the slower C–H insertion step due the steric repulsion between the methyl group and lactone ring (see Supplementary Fig. 148 and Supplementary Table 7 for DFT explanation), and its reaction at 60 °C overnight gave 4 h in only 38% yield with <5% ee (the low ee was possibly due to the racemization of the final product at high temperature, which could be initially generated in higher ee ). In addition, the naphthyl group was also tolerated for the terminating step, providing the hexacyclic fluorene 4i in 89% yield with 92% ee . In line with our previous work, the alkyl propargyl alcohol derived diazo compound 3j only led to the β-elimination product 4j after the first CAM process. The substitution pattern on the second alkyne unit (R, 4k – 4u ) was then examined, its scope was general regardless of the electronic-influence ( 4k – 4o and 4r ) or steric-effect ( 4o – 4q ) of the substituted groups on the aromatic ring, and high yields with >90% ee were obtained in these reactions. Notably, the alkyl alkyne-tethered substrate 3 s was equally reactive and offered the corresponding product in 83% yield with 68% ee . In addition, we found that the desired product 4t could be obtained in 78 yield with 84% ee in the case of the TIPS protected alkyne under the conditions with minor optimization. The terminal alkyne was also accommodated to give achiral product ( 4 u , 44%). To show the synthetic potential of this strategy, a gram-scale reaction of 3c was performed at 0.5 mol% catalyst loading (Table 3 , note b), affording 4c with comparative results (1.52 g, 89%, 94% ee ). Derivatizations of these products were also carried out to give corresponding fluorene derivatives with structural complexity, including bromination at the benzyl position, Suzuki coupling with the bromo-derivative, and saponification of the lactone (see Supplementary Methods for the synthesis of 6c , 7c , and 8c for details). Table 3 Substrates scope of carbene/alkyne metathesis terminated with asymmetric C–H functionalization a . Full size table DFT calculations on reaction 1 To support our hypothesis on enantiocontrol by the transient axial chirality, DFT calculations were carried out for reaction 1 (Tables 1 and 2 ). Substrate 1a was chosen as the model substrate. Calculation results show that the Rh(II)-catalyst provides a helical chirality environment (Fig. 2 ). Analogous acceptor-type carbene structures have been investigated by Hashimoto [62] , Charette [63] , Müller [64] , Fox [65] , Davies, and Sigman [66] , independently in their corresponding metal-carbene reactions. Initially, the dirhodium catalyst and the diazo substrate forms a complex reversibly. In the diazo-decomposition transition state, the formed chiral carbon (C*) induces the formation of the axial chirality after the leaving of N 2 gas. Based on the conformation analysis of diaryl-substituted dirhodium(II) carbene, two chiral conformers were located. DFT calculation results show that forming of the S -configuration is the favored one ( TS- S is favored over TS- R by 2.7 kcal/mol). In the structure of TS- S , remarkable π–π stacking interaction between substrate and chiral ligand can be observed. The diazo decomposition is irreversible and an activation-controlled process (not a diffusion-controlled process, see discussion in the DFT study of reaction 2 below), suggesting that the reaction will favor the S -pathway via TS- S to generate chiral rhodium(II) carbene intermediate IN- S , which has transient axial chirality because the rotation of the C–C bond is hindered by the bulky dirhodium catalysts (we did not calculate this step, but this can be well understood by the DFT study of reaction 2 below, where rotation of the axial chiral intermediate is difficult). This transitent-axial chirality is then transferred to the final product via formal C–H insertion reaction (only one transition state is available). Fig. 2: Enantioselectivity transition states of reaction 1 with 1a to 2a as example. The forming of the S -configuration product 2a is the favored one ( TS- S is favored over TS- R by 2.7 kcal/mol. Calculations at SMD(toluene)-M06L-D3/Def2TZVP//PBE-D3/Def2SVP/W06 level). Full size image DFT calculations on reaction 2 Detailed DFT calculations have also been carried out for understanding the mechanism of the key carbene/alkyne metathesis step and the transient axial chirality induced chirality transfer in this asymmetric cascade transformation (Fig. 3 ). Fig. 3: Gibbs energy profile for catalytic cascade reaction 2 with 3a to 4a as example. The discovery of carbene–Rh-dimer complex formation via ISC process in CAM process. Calculations at SMD(DCM)-M06L/6-311G(d,p)&SDD//PBE/6-31G(d)&SDD level). MECP minimum energy-crossing point. Full size image First, the nonchiral rhodium-catalyzed reaction was calculated for understanding the mechanism, especially the key carbene/alkyne metathesis step. The diazo compound 3a and Rh 2 (HCOO) 4 were chosen as a substrate and catalyst of this reaction, respectively. The potential energy surface of racemic model reaction is illustrated in Fig. 3 . The reaction starts from the complexation of Rh(II) catalyst with diazo substrate 3a , leading to the formation of IN1 (endergonic, by 4.7 kcal/mol). The complex IN1 undergoes decomposition step via TS1 , which requires an activation-free energy of 9.0 kcal/mol and is exergonic by 16.4 kcal/mol, giving rise to the corresponding Rh–carbene IN2 and liberating N 2 gas. The diazo decomposition has a computed activation-free energy of 13.7 kcal/mol and can be regarded as an activation controlled process, not diffusion-controlled process [67] . Then 5- exo - dig cyclization, via TS2 with a computed activation-free energy of 4.8 kcal/mol, converts IN2 to the zwitterionic intermediate IN3 , which is a very reactive vinyl cationic species [68] . We could not locate the corresponding intramolecular cyclopropenation transition state from IN2 , and this can be understood by considering that such reaction would generate a fused cyclopropene with high ring strain. Intermediate IN3 is subsequently converted to a more stable Rh–carbene complex IN4 via Rh-1,3-shift [69] . Our calculations indicated that this step involves an intersystem crossing (ISC) process via MECP-1 to give the triplet species, 3 IN3 , which then undergoes 1,3-Rh migration via a triplet-transition state 3 TS3 , finally giving the closed-shell singlet Rh–carbene complex IN4 . Rhodium–carbene IN4 then attacks the second tethered alkyne moiety to give the other vinyl cation intermediate IN5 . This step requires an activation-free energy of 10.1 kcal/mol. Again, IN4 converted via ISC process to a triplet species 3 IN5 with a coordinated Rh-dimer. Further coordination of Rh dimer to the carbene site via 3 TS5 (triplet diradical) to form IN6 (singlet carbene). Formal carbene C–H insertion reaction needs an activation-free energy of 21.4 kcal/mol. The final step of the catalytic cycle is releasing the product and regenerating the catalyst to continue the next catalytic cycle. The whole catalytic cycle is a downhill process and every step is easy with low activation-free energy. The final C–H insertion could be regarded as the rate-determining step of the whole catalytic process. The above computed potential energy surface provides us with a complete picture of the present cascade reaction. This mechanism has also been used to explain why the substrate 3 h has lower reactivity, mainly due to the slower C–H insertion step (see Supplementary Fig. 148 and Supplementary Table 7 for details). Of the same importance, the discovery of carbene–Rh-dimer complex formation via ISC process is significant for the future understanding of similar processes. Stereochemistry discussion for the reaction 2 The enantioselectivity of the real system was then investigated based on the above mechanistic insights. 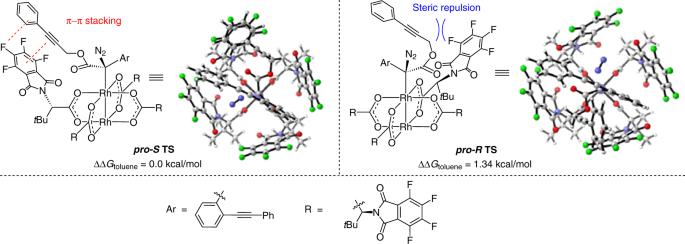Fig. 4: Enantioselectivity transition states of reaction 2 with substrate3a. Thepro-RTSis 1.34 kcal/mol higher than the correspondingpro-STS, suggesting that the experimenalee% value should be up to 80%. Calculations at SMD(toluene)-M06L-D3/Def2TZVP//PBE-D3/Def2SVP/W06 level. After formation of the complex with the diazo substrate, two possible transition states with different orientations were obtained. The pro - R TS is 1.34 kcal/mol higher than corresponding pro - S TS , suggesting that the experimental ee % value should be up to 80% (Fig. 4 ). We found that in the favored one, the phenylpropargyl group has less steric repulsion with the ligand. This transition state also benefits from weak π–π stacking interaction between phenylpropargyl group and aromatic ring of the ligand. Low-barrier intramolecular CAM process inhibits the dissociation of the catalyst and other side reactions, thus this initially formed transient axial chirality in the metal-carbene intermediate that controlled the following asymmetric transfer processes, and enabling the stereospecificity chirality transfer in the final formal C–H insertion step via an axial-to-point chirality transfer model [70] . According to the above results, the mechanistic proposal of this fluorene ring formation using chiral dirhodium as a catalyst is depicted in Fig. 5 . In the initial step, Rh(II)-mediated decomposition of diazo compound 3a generated the first chiral carbene intermediate I with axial chirality due to the hindered rotation of the congested geometry. Followed by a dual-carbene/alkyne metathesis process to form the third axial chirality–carbene-intermediate III via the second one II . Finally, the catalytic cycle is finished by a selective C(sp 2 )-H insertion with the axial chirality transfer to the carbon chirality center via an axial-induced-point chirality transfer model. Fig. 4: Enantioselectivity transition states of reaction 2 with substrate 3a . The pro - R TS is 1.34 kcal/mol higher than the corresponding pro - S TS , suggesting that the experimenal ee % value should be up to 80%. Calculations at SMD(toluene)-M06L-D3/Def2TZVP//PBE-D3/Def2SVP/W06 level. Full size image Fig. 5: Overview of the catalytic cycle. The dual-carbene/alkyne metathesis process through the formation of the carbene intermediates with axial chirality. Full size image Considering the C–H insertion is the rate-determine step in this tandem reaction, we calculated the barrier of C–H insertion and rotation of c -INT3 in real system (Fig. 6 ), the barrier of final C–H insertion reaction is 23.7 kcal/mol, which is consistent with the experimental result. The rotation barrier here is 13.4 kcal/mol higher than C–H insertion reaction, so the chiral transfer is complete in this step and the enantioselective determining step is not C–H insertion step here. For other two optimized key structures of I and II in real system, see Supplementary Fig. 152 for details. Fig. 6: Rotation vs Csp 2 –H insertion. The calculated rotation barrier of c -INT3 is 13.4 kcal/mol higher than C–H insertion reaction. Full size image In summary, we have reported a transient axial-chirality transfer strategy for asymmetric reaction, which takes advantage of the point chirality of the dirhodium catalyst that can be transferred to a Rh–carbene intermediate with transient axial chirality due to the hindered rotation introduced by the bulky catalyst. This transient axial-chirality can ensure the high stereoselectivity in the followed formal Csp 2 –H insertion reaction. We also generalized this strategy for asymmetric cascade reaction via dual-carbene/alkyne metathesis process. DFT calculations reveal the π–π stacking predominant chiral recognition pattern and the unique axial-to-point chirality transfer. Also detailed mechanistic study of the reaction mechanism of two reactions have been investigated, finding that intersystem crossing (ISC) process have been encountered in generating Rh–carbene species. Further applications of this transient axial-chirality transfer concept could be envisioned for other asymmetric reactions. General methods See Supplementary Methods for further details. Typical procedure for the direct asymmetric C–H functionalization reaction To a 10-mL oven-dried vial containing a magnetic stirring bar, diazo compound 1 (0.2 mmol), and 4 Å MS (100 mg) in TBME (1.0 mL) and Rh 2 (S-TFPTTL) 4 (3.0 mg, 1.0 mol%) was added as a solution in TBME (1.0 mL) via a syringe pump over 40 min under argon atmosphere at room temperature. 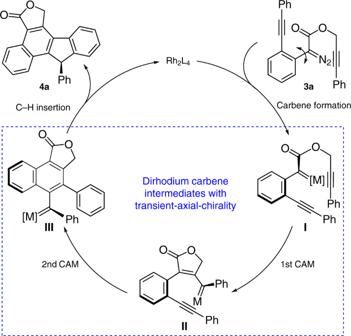Fig. 5: Overview of the catalytic cycle. The dual-carbene/alkyne metathesis process through the formation of the carbene intermediates with axial chirality. 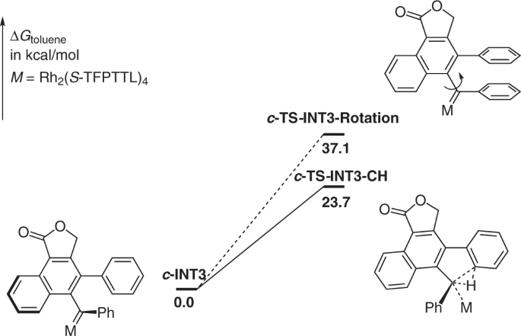Fig. 6: Rotation vs Csp2–H insertion. The calculated rotation barrier ofc-INT3is 13.4 kcal/mol higher than C–H insertion reaction. After addition, the reaction mixture was stirred for additional 1–5 h, as indicated, and then purified by column chromatography on silica gel without any additional treatment (hexanes: DCM = 20:1 to 10:1) to give the desired 9-aryl fluorene products 2 . Typical procedure for the asymmetric cascade reaction To a 10-mL oven-dried vial containing a magnetic stirring bar, diazo compound 3 (0.2 mmol), and 4 Å MS (100 mg) in TBME (1.0 mL) and Rh 2 (S-TFPTTL) 4 (3.0 mg, 1.0 mol%) was added as a solution in TBME (1.0 mL) via a syringe pump over 40 min under argon atmosphere at 40 °C. After addition, the reaction mixture was stirred for additional 20 min, and then purified by column chromatography on silica gel without any additional treatment (hexanes: DCM = 2:1 to 1:1) to give the desired polycyclic products 4 .